Retinoic acid signalling regulates the development of tonotopically patterned hair cells in the chicken cochlea Precise frequency discrimination is a hallmark of auditory function in birds and mammals and is required for distinguishing similar sounding words, like ‘bat,’ ‘cat’ and ‘hat.’ In the cochlea, tuning and spectral separation result from longitudinal differences in basilar membrane stiffness and numerous individual gradations in sensory hair cell phenotypes, but it is unknown what patterns the phenotypes. Here we used RNA-seq to compare transcriptomes from proximal, middle and distal regions of the embryonic chicken cochlea, and found opposing longitudinal gradients of expression for retinoic acid (RA)-synthesizing and degrading enzymes. In vitro experiments showed that RA is necessary and sufficient to induce the development of distal-like hair cell phenotypes and promotes expression of the actin-crosslinking proteins, Espin and Fscn2. These and other findings highlight a role for RA signalling in patterning the development of a longitudinal gradient of frequency-tuned hair cell phenotypes in the cochlea. In the elongated cochleae of reptiles, birds and mammals, sound stimulation causes peaks of vibration at different longitudinal positions extending from the high-frequency-sensitive proximal (tympanic) end to the low-frequency-sensitive distal end [1] . In reptiles and birds, auditory tuning stems in large measure from the electrical resonance properties of hair cells (HCs), which differ with the expression and response kinetics of large-conductance Ca 2+ -activated BK channels that vary along the cochlea’s length [2] , [3] , [4] , [5] , [6] . HCs in these cochleae also exhibit striking differences in the number and length of actin-filled stereocilia that make up their apical mechanoreceptive hair bundles. In the auditory sensory epithelium of the chicken basilar papilla (BP), hair bundles at the proximal, high-frequency-sensitive end contain >250 stereocilia that reach a maximum length of 1.5 μm, while those in the distal, low-frequency-sensitive end contain <50 stereocilia with a maximum length of 5.5 μm ( Fig. 1a–c ) [7] , [8] . At locations between those ends, the number and length of the tallest stereocilia vary progressively along the tonotopic axis. Similar spatial gradients occur in the mammalian cochlea [9] , [10] . 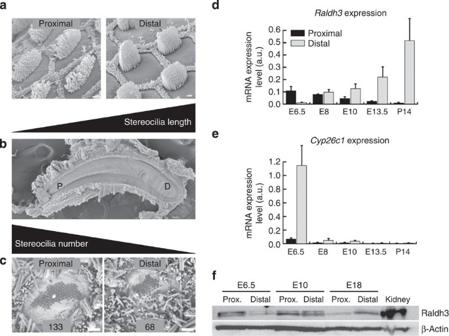Figure 1: Gradients of HC phenotypes develop along the longitudinal axis of the chicken cochlea. (a) Scanning electron micrographs (SEM) showing short sensory hair bundles that project from the apical surfaces of HCs at the proximal end of the BP sensory epithelium and tall bundles of HCs at the distal end. The HCs are surrounded by honeycomb-like patterns comprising the microvilli-covered surfaces of SCs. (b) Low-magnification SEM image showing the sickle-shaped BP, which is narrow proximally (P) and broad distally (D). (c) SEM images of HCs that formedin vitroin E6.5 BPs cultured in control medium for 7 days. The hair bundles in these micrographs were broken off so that the bases of the individual stereocilia could be counted, which showed that the HCs at the proximal end of cultured BPs contained more stereocilia than HCs at the distal end as do HCs that developin ovo. (d) Histogram showing developmental changes in mRNA levels for the RA synthetic enzyme,Raldh3, in the proximal (dark bars) and distal (light bars) halves of BP as measured in qRT–PCR. At E6.5,Raldh3is expressed in a proximal-to-distal gradient, which reverses and becomes a strengthening distal-to-proximal gradient at later stages of cochlear development. (e) Histogram of mRNA levels for the RA-catabolizing enzyme,Cyp26c1, measured from qRT–PCR. At E6.5,Cyp26c1is expressed in a distal-to-proximal gradient, but mRNA expression declines to barely detectable levels at later developmental stages. Graphs show the mean mRNA expression levels (arbitrary units) measured in the proximal and distal regions ±s.e.m. (f) Representative western blot for of Raldh3 and β-actin protein in the proximal and distal halves of E6.5, E10 and E18 cochlea (n=3). E18 kidney was used as a positive control tissue and β-actin was used as a loading control. At E6.5, Raldh3 was enriched 4.43-fold in the proximal BP compared with the distal BP, but the relative protein levels reverse as development progressed, with 3.87-fold more Raldh3 protein in the distal BP than in proximal BP at E18. Levels were approximately equivalent in the proximal and distal E10 BPs. Scale bars, 1 μm. Figure 1: Gradients of HC phenotypes develop along the longitudinal axis of the chicken cochlea. ( a ) Scanning electron micrographs (SEM) showing short sensory hair bundles that project from the apical surfaces of HCs at the proximal end of the BP sensory epithelium and tall bundles of HCs at the distal end. The HCs are surrounded by honeycomb-like patterns comprising the microvilli-covered surfaces of SCs. ( b ) Low-magnification SEM image showing the sickle-shaped BP, which is narrow proximally (P) and broad distally (D). ( c ) SEM images of HCs that formed in vitro in E6.5 BPs cultured in control medium for 7 days. The hair bundles in these micrographs were broken off so that the bases of the individual stereocilia could be counted, which showed that the HCs at the proximal end of cultured BPs contained more stereocilia than HCs at the distal end as do HCs that develop in ovo . ( d ) Histogram showing developmental changes in mRNA levels for the RA synthetic enzyme, Raldh3 , in the proximal (dark bars) and distal (light bars) halves of BP as measured in qRT–PCR. At E6.5, Raldh3 is expressed in a proximal-to-distal gradient, which reverses and becomes a strengthening distal-to-proximal gradient at later stages of cochlear development. ( e ) Histogram of mRNA levels for the RA-catabolizing enzyme, Cyp26c1 , measured from qRT–PCR. At E6.5, Cyp26c1 is expressed in a distal-to-proximal gradient, but mRNA expression declines to barely detectable levels at later developmental stages. Graphs show the mean mRNA expression levels (arbitrary units) measured in the proximal and distal regions ±s.e.m. ( f ) Representative western blot for of Raldh3 and β-actin protein in the proximal and distal halves of E6.5, E10 and E18 cochlea ( n =3). E18 kidney was used as a positive control tissue and β-actin was used as a loading control. At E6.5, Raldh3 was enriched 4.43-fold in the proximal BP compared with the distal BP, but the relative protein levels reverse as development progressed, with 3.87-fold more Raldh3 protein in the distal BP than in proximal BP at E18. Levels were approximately equivalent in the proximal and distal E10 BPs. Scale bars, 1 μm. Full size image The tonotopic (longitudinally frequency-tuned) gradients in HC phenotypes form even in cochleae derived from otocysts that have been denervated after 3 days of incubation (E3) [11] , [12] . Yet, the signals that pattern the phenotypes are unknown. Hypothesizing that morphogen levels might differ as the gradient of phenotypes developed, we sequenced the transcriptomes of the proximal, middle and distal thirds of the chicken cochlea at E6.5, when post-mitotic HCs first form [13] . Of >1,000 differentially expressed genes, one involved in the synthesis of RA ( Raldh3 ) and one involved in its degradation ( Cyp26c1 ) displayed opposing longitudinal gradients of expression. In the developing retina and hindbrain, morphogenetic gradients of RA are established and confined between regions of high Raldh and Cyp26 expression [14] , [15] , and such gradients play crucial roles in patterning the anterior–posterior axis of the early embryo, the spinal cord and the early otocyst (E2–E3) [15] , [16] , [17] , [18] . To investigate whether RA plays a role in patterning the gradient of HC phenotypes, we developed an in vitro model that supports cochlear development, free from potentially confounding influences of most neighbouring tissues. Using that model, we found that proximal HCs acquired distal-like phenotypes when they differentiated in the presence of exogenous RA, and distal HCs developed proximal-like phenotypes when they differentiated in the presence of RA antagonists. These, and other findings, show that RA signalling is both necessary and sufficient for the specification of important features of distal-like HC phenotypes. RNA-seq analysis We isolated mRNA from proximal, middle and distal sections of E6.5 BPs for Illumina sequence analysis aimed at identifying gradients of gene expression along the tonotopic axis. The data sets for all three regions comprise >10,000 detectably expressed genes and are available in Supplementary Data 1 . Raw sequences have been submitted to NCBI GEO (accession number GSE56888). In addition to the developing BP, the avian cochlear duct also houses the lagena, an otolithic organ, which we were not able to distinguish or separate from the BP at E6.5. Therefore, the sequencing results from the distal E6.5 BP may contain lagena-expressed genes. To identify transcripts that might reveal gradients of morphogen expression, we applied three filters. First, we selected only genes that exhibited ⩾ 2-fold change between the proximal and distal regions. We then eliminated genes that failed to pass a ⩾ 0.5 RPKM (reads per kilobase of exon per million fragments mapped; ref. 19 ) abundance threshold in either region, and we removed genes that exhibited peaks or valleys of expression in the middle of the BP. The resulting data set includes 1,254 genes that exhibit gradients of transcript abundance between the two ends of the BP. These are listed in Supplementary Data 2 , along with their abundance profiles and some functional annotations. Interestingly, this list is heavily biased towards genes that show much higher transcript abundance in the proximal BP (1,104 genes) than in the distal BP (150 genes). Among these results are genes in seven signalling pathways that play a role in inner ear development: Retinoic acid (RA), Hedgehog, FGF, Wnt, Notch, TGF-β and IGF signalling. Our RNA-seq results suggested the presence of a source and sink for RA at opposing ends of the BP at E6.5, as indicated by the high expression of Raldh3 in the proximal BP and the high expression of Cyp26c1 in the distal BP ( Table 1 ). Retinaldehyde dehydrogenase 3, Raldh3 (also Aldh1a3), is one of three dehydrogenases that catalyse retinaldehyde oxidation to produce RA, and is required for patterning the retina [20] . Cyp26c1 is one of three cytochrome p450 (Cyp26) enzymes that regulate RA signalling by catalysing RA degradation [14] . The RNA-seq results also show that RAR α and RXR γ, which encode two retinoid receptors, and Crabp1 , which encodes the cellular retinoic acid-binding protein 1, are expressed at levels that are respectively 2.2-fold, 3.1-fold and 5-fold higher proximally than distally. Although Crabp1 function is not completely resolved, evidence suggests it may have a role in binding and sequestering RA in the cytoplasm [21] . Table 1 Expression levels in the E6.5 chicken BP for a subset of expressed genes that are involved in RA signalling. Full size table Additional evidence for the involvement of RA was provided by network analysis, through which we identified 112 transcription-factor-encoding genes that are expressed in gradients along the BP ( Supplementary Data 3 ). The data in Supplementary Data 2 were uploaded to g:Profiler and analysed by gene group functional profiling [22] , which showed literature-supported interactions among 75 genes that are differentially expressed along the BP, including RAR α and RXR γ and 21 additional transcription factor genes ( Supplementary Fig. 1 ). Among these are RA-responsive genes, such as Hoxd4 , and the nuclear hormone receptor genes for Thyroid Hormone Receptor β ( THRB ) and the Peroxisome Proliferator-Activated Receptor ( PPAR ). Network analysis also identified the Androgen Receptor ( AR ), which is known to have inhibitory interactions with RXR family members [23] . In the BP, AR is expressed in a distally high gradient, opposite to the gradient of RXR γ expression. Supplementary Data 2 was also analysed with the Ingenuity Pathway Analysis (IPA) Upstream Regulator analytic to search out candidate upstream transcriptional regulators that might be involved in establishing gene expression differences between the proximal and distal parts of the BP. All- trans retinoic acid (aka tretinoin) was the most significant candidate detected (by absolute activation z score, Supplementary Table 1 ), further implicating RA as a candidate patterning signal. The gradients of RA pathway genes reverse as the BP develops To validate the RNA-seq results and determine whether expression levels change between E6.5 and P14, we isolated samples from the proximal and distal ends of BPs over the course of development and performed qRT–PCR ( Fig. 1d,e ). The PCR results confirmed the presence of reciprocal Raldh3 and Cyp26c1 expression gradients at E6.5 consistent with higher levels of RA at the proximal end of the BP. However, analysis at later developmental time points revealed marked changes in expression. Raldh3 expression increased dramatically in the distal BP at E8, and continued to increase through P14. At the same time points expression in the proximal BP decreased such that by E10 the gradient of Raldh3 had reversed and was higher at the distal end. At the same time points Cyp26c1 expression declined to barely detectable levels ( Fig. 1d,e ). To confirm the qPCR data, we performed western blots for Raldh3 protein levels in tissue isolated from distal and proximal regions of the BP at E6.5, E10 and E18. Results indicated that Raldh3 protein is expressed at 4.43-fold greater levels in proximal versus distal BP at E6.5 ( Fig. 1f ). But by E10 proximal and distal samples appear equivalent. Finally, at E18 Raldh3 is expressed at 3.87-fold greater levels in the distal BP. These data are consistent with the qPCR data and confirm a marked switch in expression of Raldh3 between E6.5 and E10. To determine which cells within the BP express Raldh3, immunohistochemistry was performed on whole-mount BPs. At E8, Raldh3 was strongly expressed in presumptive supporting cells (SCs), while HCs were negative ( Fig. 2 ). At E10, however, Raldh3 appeared to be expressed in both SCs and HCs. In addition, consistent with the qPCR and western results, the overall level of Raldh3 appeared higher in the distal region of the BP. By E18, Raldh3 was expressed predominately in HCs in both the proximal and distal ends of the BP. We hypothesize that the reversal of the longitudinal gradient of Raldh3 mRNA expression that occurs between E6.5 and E10 is linked to the change from expression of Raldh3 protein in SCs to expression that is predominantly in HCs. 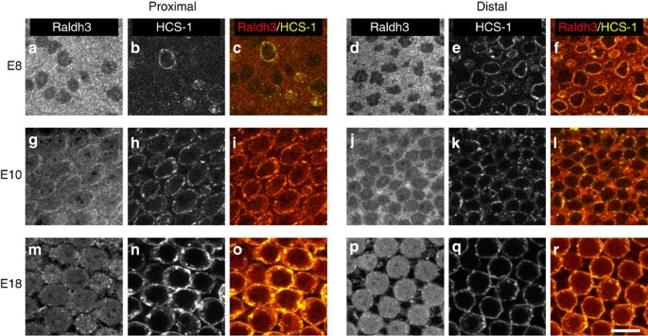Figure 2: Raldh3 predominately expressed in SCs early in development, but HCs become the predominant expressers at later stages. Representative images from immunolabelling using antibodies to Raldh3 (a,d,g,j,m,p) and HCS-1 (otoferlin) (b,e,h,k,n,q) in the proximal (left) and distal (right) regions of the BPs from embryos at E8 (a–f), E10 (g–l) and E18 (m–r). The grey scale images in the far left on each side show Raldh3 immunofluorescence. Middle panel images show HCS-1 immunofluorescence, and images in the far right panels on each side show the merged immunofluorescence from Raldh3 (red) and HCS-1 (yellow). At E8, the antibody to Raldh3 most strongly labelled the SCs, which are negative for HCS-1, but labelling in HCs increased at E10, and at E18, Raldh3 was predominantly expressed by HCs. Each immunolabelling experiment was independently replicated three times. Scale bar, 10 μm. Figure 2: Raldh3 predominately expressed in SCs early in development, but HCs become the predominant expressers at later stages. Representative images from immunolabelling using antibodies to Raldh3 ( a , d , g , j , m , p ) and HCS-1 (otoferlin) ( b , e , h , k , n , q ) in the proximal (left) and distal (right) regions of the BPs from embryos at E8 ( a – f ), E10 ( g – l ) and E18 ( m – r ). The grey scale images in the far left on each side show Raldh3 immunofluorescence. Middle panel images show HCS-1 immunofluorescence, and images in the far right panels on each side show the merged immunofluorescence from Raldh3 (red) and HCS-1 (yellow). At E8, the antibody to Raldh3 most strongly labelled the SCs, which are negative for HCS-1, but labelling in HCs increased at E10, and at E18, Raldh3 was predominantly expressed by HCs. Each immunolabelling experiment was independently replicated three times. Scale bar, 10 μm. Full size image The longitudinal gradient in the number of stereocilia per HC becomes evident by E10.5 and the developing gradient in the height of the hair bundles becomes evident by E12 (refs 24 , 25 , 26 , 27 ). Consistent with the possibility that high distal RA promotes distal-like hair bundle phenotypes, the reversal of the Raldh3 expression gradient shown in the qRT–PCR and western blot data occurs during the stages when the longitudinal gradients of HC phenotypes first become evident. To confirm that expression levels of Raldh3 correspond with actual levels of RA, we dissected E10 BPs, then separately cultured their proximal and distal halves on RA reporter cells [28] , [29] . E10 retina and media that contained either 5 nM or 100 nM RA were used as positive controls. Few reporter cells in the vicinity of the proximal halves were positive for the blue LacZ signal, but many were positive in the vicinity of the distal halves ( Fig. 3 ). These results demonstrate that by E10, the levels of Raldh3 mRNA, Raldh3 protein and soluble RA are higher in the distal BP than in the proximal BP. 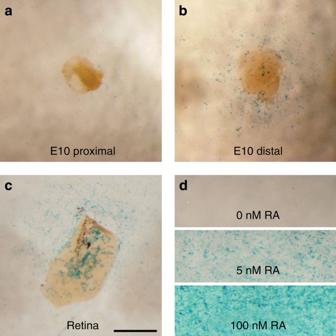Figure 3: Soluble RA levels are higher in the distal half of the BPs at E10. Bright-field images ofLacZexpression in RA reporter cells (F9-RARE-LacZ) that were co-cultured with proximal (a) and distal halves (b) from the same E10 BP. Many cells in the vicinity of the distal samples were positive for the blueLacZsignal while few in the vicinity of the proximal sample were. (c) E10 retinal tissue was used as a tissue control. (d) As pharmacological controls, reporter cells in separate wells were exposed to 0 nM, 5 nM and 100 nM RA. Scale bar, 1 mm. Figure 3: Soluble RA levels are higher in the distal half of the BPs at E10. Bright-field images of LacZ expression in RA reporter cells (F9-RARE-LacZ) that were co-cultured with proximal ( a ) and distal halves ( b ) from the same E10 BP. Many cells in the vicinity of the distal samples were positive for the blue LacZ signal while few in the vicinity of the proximal sample were. ( c ) E10 retinal tissue was used as a tissue control. ( d ) As pharmacological controls, reporter cells in separate wells were exposed to 0 nM, 5 nM and 100 nM RA. Scale bar, 1 mm. Full size image The cellular effects of RA are mediated through members of the RAR and RXR nuclear receptor families, which form functional heterodimers [18] . Our sequencing results from the E6.5 BP showed significant expression of two RARs, RAR α and RAR β, but only one of the RXR nuclear receptors, RXR γ. Like the RNA-seq analysis, qRT–PCR showed that RXR γ is expressed in a proximal-high gradient at E6.5, but the RXR γ expression gradient reverses and becomes a distal-high gradient at E8 and E10, contemporaneous with the reversal of the Raldh3 expression gradient ( Fig. 4a ). Throughout the stages of development that we assessed, the potential RXR γ dimerization partners, RAR α and RAR β, were expressed at essentially equivalent levels in both ends of the BP ( Fig. 4c ). 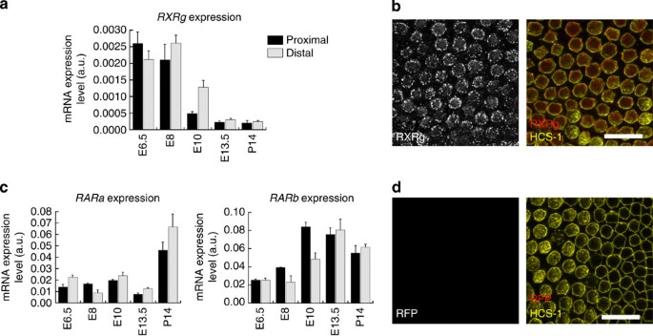Figure 4: RA nuclear receptor expression in the developing cochlea. (a) Histogram showingRXRγ mRNA expression levels measured from qRT–PCR of the proximal (dark bars) and distal (light bars) regions of E6.5, E8, E10, E13.5 and P14 BPs. RXRγ becomes expressed in a distal-to-proximal gradient at E8 and E10. (b) Representative confocal micrograph showing RXRγ (red) and HCS-1 (yellow) immunofluorescence in E18 BPs. Left panel shows grey scale from RXRγ alone and the right panel shows the merged immunofluorescence from RXRγ (red) and HCS-1 (yellow). RXRγ immunofluorescence is observable within the HCS-1-positive HCs. (c) Histograms showing mRNA expression levels forRARα andRARβ in proximal (dark bars) and distal (light bars) regions of E6.5, E8, E10, E13.5 and P14 BPs. Throughout the stages of development assessed, these nuclear receptors were expressed in both ends of the BP. (d) Representative negative control immunofluorescence with red fluorescence protein (RFP) antibody. Left panel shows grey scale from RFP alone and right panel shows immunofluorescence from RFP (red) and HCS-1 (yellow). Each immunolabelling experiment was independently replicated three times. Graphs show the mean mRNA expression levels (arbitrary units) measured in the proximal and distal regions ±s.e.m. Scale bars, 20 μm. Figure 4: RA nuclear receptor expression in the developing cochlea. ( a ) Histogram showing RXR γ mRNA expression levels measured from qRT–PCR of the proximal (dark bars) and distal (light bars) regions of E6.5, E8, E10, E13.5 and P14 BPs. RXRγ becomes expressed in a distal-to-proximal gradient at E8 and E10. ( b ) Representative confocal micrograph showing RXRγ (red) and HCS-1 (yellow) immunofluorescence in E18 BPs. Left panel shows grey scale from RXRγ alone and the right panel shows the merged immunofluorescence from RXRγ (red) and HCS-1 (yellow). RXRγ immunofluorescence is observable within the HCS-1-positive HCs. ( c ) Histograms showing mRNA expression levels for RAR α and RAR β in proximal (dark bars) and distal (light bars) regions of E6.5, E8, E10, E13.5 and P14 BPs. Throughout the stages of development assessed, these nuclear receptors were expressed in both ends of the BP. ( d ) Representative negative control immunofluorescence with red fluorescence protein (RFP) antibody. Left panel shows grey scale from RFP alone and right panel shows immunofluorescence from RFP (red) and HCS-1 (yellow). Each immunolabelling experiment was independently replicated three times. Graphs show the mean mRNA expression levels (arbitrary units) measured in the proximal and distal regions ±s.e.m. Scale bars, 20 μm. Full size image HCs in the developing mouse cochlea are known to express RA receptors and are responsive to RA signals [30] . In the BPs of E18 chickens, immunolabelling with an antibody against RXRγ clearly labelled HCs, while a negative control antibody (to Red Fluorescent Protein) produced no labelling ( Fig. 4b,d ). Since our results show that HCs express the RA-synthesizing enzyme, Raldh3, and the nuclear receptor, RXRγ, RA may have autocrine signalling effects in these sensory cells. The release of soluble RA that was detected by reporter cells growing in the vicinity of cultured BP tissues ( Fig. 3 ) is also consistent with RA-mediated paracrine signalling. Thus, autocrine or paracrine signalling may both potentially play roles during BP development, perhaps at different stages. RA signalling induces distal-like HC phenotype formation To determine whether the distally high RA gradient influences the patterning of HC phenotypes along the tonotopic axis, we cultured E6.5 BPs for 7 days, which allowed the HCs to progress through differentiation of their location-specific phenotypes. Experimental cultures were maintained in medium supplemented with 500 nM all- trans -retinoic acid (hereafter RA) and control cultures were maintained in medium containing vehicle alone. We then fixed the cultures and assessed the phenotypic characteristics of the HCs that developed near the proximal and distal ends. The resulting quantified HC phenotypes and number of BPs analysed for each experimental treatment (control, RA or the RA antagonist citral) are shown in Table 2 . In the control cultures, proximal HCs developed more stereocilia than distal HCs, paralleling the gradient that forms in ovo ( Fig. 5c ). BPs cultured with RA also developed a gradient of stereocilia number, but with fewer stereocilia per cell. HCs in the proximal end of RA-treated BPs developed 68.6% of the number of stereocilia that formed in proximal HCs of control cultures, while distal HCs formed 53.5% of the number in the distal HCs of controls ( Fig. 5c ; P <0.05 for each, n BPs =6; except when indicated, P -values were from one-way analysis of variance (ANOVA) with Newman–Keuls post-test). Table 2 Quantified HC phenotypes. 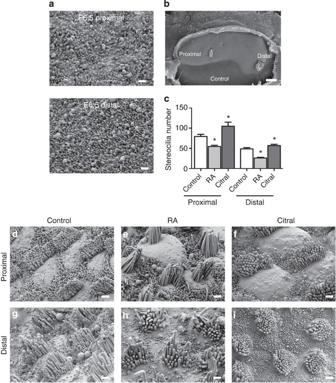Figure 5: Modulating retinoic acid signalling disrupts tonotopic gradient of stereocilia number. (a) Representative scanning electron micrograph of proximal and distal regions of E6.5 BPs. There is no apparent stereocilia formation at this stage in either region. (b) Micrograph of E6.5 BP explant cultured 7 days in control medium. Proximal and distal regions are indicated. (c) Quantification of the number of stereocilia that formed in the proximal and distal regions of treated BPs. HCs form fewer stereocilia in both proximal and distal regions in RA-treated BPs. HCs form more stereocilia in proximal and distal regions of citral-treated BPs. *P<0.05; one-way ANOVA with Newman–Keuls post-test. (d–i) Representative micrographs of HCs that form in the proximal and distal regions of E6.5 BPs cultured for 7 days in control media (d,g), with RA (e,h), or with citral (f,i). Total number of BPs analysed aren=8 for control;n=6 for RA;n=8 for citral. Graph shows mean±s.e.m. Scale bars inb, 100 μm;a,c–h, 1 μm. Full size table Figure 5: Modulating retinoic acid signalling disrupts tonotopic gradient of stereocilia number. ( a ) Representative scanning electron micrograph of proximal and distal regions of E6.5 BPs. There is no apparent stereocilia formation at this stage in either region. ( b ) Micrograph of E6.5 BP explant cultured 7 days in control medium. Proximal and distal regions are indicated. ( c ) Quantification of the number of stereocilia that formed in the proximal and distal regions of treated BPs. HCs form fewer stereocilia in both proximal and distal regions in RA-treated BPs. HCs form more stereocilia in proximal and distal regions of citral-treated BPs. * P <0.05; one-way ANOVA with Newman–Keuls post-test. ( d – i ) Representative micrographs of HCs that form in the proximal and distal regions of E6.5 BPs cultured for 7 days in control media ( d , g ), with RA ( e , h ), or with citral ( f , i ). Total number of BPs analysed are n= 8 for control; n =6 for RA; n= 8 for citral. Graph shows mean±s.e.m. Scale bars in b , 100 μm; a , c – h , 1 μm. Full size image Next we investigated whether exogenous RA affected the size of the luminal surfaces of the HCs. In control cultures, proximal HCs formed larger luminal surfaces than distal HCs ( Fig. 6i ). In contrast, proximal HCs in BPs that were cultured with added RA developed luminal surfaces that reached just 52.2% of the size formed in control ( P <0.05, n BPs =20). All of these results are consistent with a role for the E8–E10 distal-to-proximal gradient of RA in the specification of location-specific HC phenotypes along the BP. 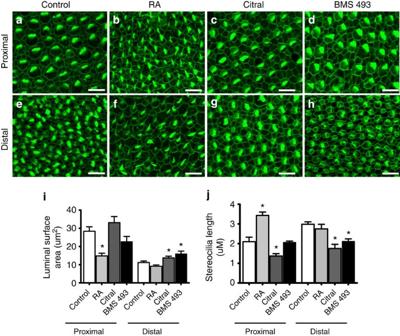Figure 6: Modulating RA disrupts tonotopic gradients of hair bundle heights and HC luminal surface area. Example micrographs of HCs that form in the proximal and distal regions of E6.5 BPs cultured 7 days with control media (a,e), RA (b,f), citral (c,g) or BMS 493 (d,h). Hair bundle heights were analysed from confocal micrographs using Imaris 3D software (Bitplane). (i) Quantification of HC luminal surface areas that formed in the proximal and distal regions of treated BPs measured using ImageJ from confocal maximum projections. HCs that formed in the proximal region of BPs treated with RA developed smaller luminal surfaces than HCs that formed in the proximal region of control BPs. Further, HCs that formed in the distal region of BMS 493 and citral-treated cochlea developed larger luminal surfaces than HCs that formed in the distal regions of control BPs. Total number of BPs analysed aren=15 for control;n=20 for RA;n=12 for citral;n=6 for BMS 493 treatments. (j) Quantification of the maximal hair bundle heights that formed in the proximal and distal regions of treated BPs. Proximal HCs formed longer hair bundles in RA-treated BPs compared with control proximal HCs. In addition, citral treatments lead to significantly shorter hair bundles in both proximal and distal regions compared with controls. BPs treated with BMS 493 developed shorter hair bundles in the distal region (nBPs=6). *P<0.05; one-way ANOVA with Newman–Keuls post-test. Total number of BPs analysed aren=8 for control;n=9 for RA;n=8 for citral;n=6 for BMS 493 treatments. Graph shows mean±s.e.m. Scale bars, 10 μm. Figure 6: Modulating RA disrupts tonotopic gradients of hair bundle heights and HC luminal surface area. Example micrographs of HCs that form in the proximal and distal regions of E6.5 BPs cultured 7 days with control media ( a , e ), RA ( b , f ), citral ( c , g ) or BMS 493 ( d , h ). Hair bundle heights were analysed from confocal micrographs using Imaris 3D software (Bitplane). ( i ) Quantification of HC luminal surface areas that formed in the proximal and distal regions of treated BPs measured using ImageJ from confocal maximum projections. HCs that formed in the proximal region of BPs treated with RA developed smaller luminal surfaces than HCs that formed in the proximal region of control BPs. Further, HCs that formed in the distal region of BMS 493 and citral-treated cochlea developed larger luminal surfaces than HCs that formed in the distal regions of control BPs. Total number of BPs analysed are n =15 for control; n =20 for RA; n =12 for citral; n =6 for BMS 493 treatments. ( j ) Quantification of the maximal hair bundle heights that formed in the proximal and distal regions of treated BPs. Proximal HCs formed longer hair bundles in RA-treated BPs compared with control proximal HCs. In addition, citral treatments lead to significantly shorter hair bundles in both proximal and distal regions compared with controls. BPs treated with BMS 493 developed shorter hair bundles in the distal region ( n BPs =6). * P <0.05; one-way ANOVA with Newman–Keuls post-test. Total number of BPs analysed are n= 8 for control; n =9 for RA; n= 8 for citral; n =6 for BMS 493 treatments. Graph shows mean±s.e.m. Scale bars, 10 μm. Full size image Finally, we used confocal micrographs and 3D images produced using Imaris software (Bitplane) to make preliminary measurements of hair bundle heights in BPs cultured under different conditions. In control cultures, proximal HCs formed shorter hair bundles than distal HCs ( Fig. 6j ). In contrast, proximal HCs in BPs that were cultured with added RA developed hair bundles that were 62.6% longer than those of proximal HCs in the controls ( P <0.05, n BPs =9). Surprisingly, the direction of the longitudinal gradient of hair bundle heights reversed in BPs that were cultured with exogenous RA. Proximal HCs developed significantly longer hair bundles than distal HCs in RA-treated BPs ( P <0.05, Student’s t- test). Taken together, these results indicate that RA signalling is sufficient to induce distal-like HC phenotypes, even in the proximal BP. Since z axis resolution is severely limited in light microscopy, we used scanning electron microscopy (SEM) as an independent, higher-resolution method for measuring hair bundle heights. For this, we sampled different locations along the length of BPs that were fixed and processed for SEM after culturing for 7 days in media containing 500 nM RA or vehicle alone. Although fixation and processing for SEM lead to significant shrinkage errors over measurements in unfixed hydrated tissue [31] , SEM provides high-resolution measurements for assessing relative bundle height differences along the BP’s length. At each location sampled we captured SEM images in stereo pairs and then measured hair bundle heights using a double-blind approach. Calculations from this unbiased and higher-resolution measurement method showed that proximal HCs in the RA-treated BPs grew hair bundles that were more than two times the height (128% higher) than those in control BP cultures ( P< 0.05, n BPs =4, Fig. 7b ). Thus, low-resolution 3D confocal imaging and higher-resolution stereoimaging measurements from SEM were consistent and supported the same conclusions. 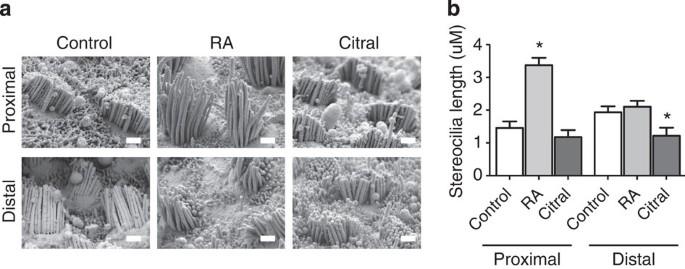Figure 7: SEM stereoimaging validation of hair bundle heights measurements. (a) Representative micrographs of E6.5 BPs that were cultured for 7 days in control medium or media supplemented with RA or citral. HCs were viewed from behind the longest stereocilia and stereopair images were taken from four neighbouring fields at a distance of ~18% of the total length of the BP away from the proximal and distal ends (nBPs=4 for each treatment). Micrographs were blinded and hair bundle heights were then measured from stereopair images. (b) Quantifications of the stereocilia lengths that were measured from stereopair SEM images taken at 15,000 X. Proximal HCs were taller in the RA-treated BPs compared with control BPs: 3.37±0.22 μm versus 1.46±0.20 μm, respectively. Further, distal HCs were shorter in the BPs treated with citral compared with controls: 1.21±0.25 μm versus 1.93±0.19 μm, respectively. *P<0.05; one-way ANOVA with Newman–Keuls post-test. Graph shows the mean hair bundle height measured in the proximal and distal regions ±s.e.m. Scale bars, 1 μm. Figure 7: SEM stereoimaging validation of hair bundle heights measurements. ( a ) Representative micrographs of E6.5 BPs that were cultured for 7 days in control medium or media supplemented with RA or citral. HCs were viewed from behind the longest stereocilia and stereopair images were taken from four neighbouring fields at a distance of ~18% of the total length of the BP away from the proximal and distal ends ( n BPs =4 for each treatment). Micrographs were blinded and hair bundle heights were then measured from stereopair images. ( b ) Quantifications of the stereocilia lengths that were measured from stereopair SEM images taken at 15,000 X. Proximal HCs were taller in the RA-treated BPs compared with control BPs: 3.37±0.22 μm versus 1.46±0.20 μm, respectively. Further, distal HCs were shorter in the BPs treated with citral compared with controls: 1.21±0.25 μm versus 1.93±0.19 μm, respectively. * P <0.05; one-way ANOVA with Newman–Keuls post-test. Graph shows the mean hair bundle height measured in the proximal and distal regions ±s.e.m. Scale bars, 1 μm. Full size image To determine whether RA signalling is necessary for the formation of distal-like HC phenotypes, we cultured E6.5 BPs for 7 days in medium containing 5 μM citral, a competitive inhibitor of Raldhs that has been used to block RA synthesis in multiple systems, including the mouse cochlea and retina [30] , [32] , [33] , [34] , [35] . HCs that developed in the citral-treated BPs formed bundles with significantly more stereocilia regardless of whether they were located in the distal or proximal region of the BP ( P <0.05 for each, n BPs =8, Fig. 5c ). However when presented as a percentage change, the effect was more pronounced in the proximal region where the increase in stereocilia was 31.9% over control as compared with an increase of 17.1% over control in the distal region. Distal HCs that differentiated in the presence of citral developed luminal surface that were 23% larger than their counterparts in controls ( P <0.05, n BPs =12, Fig. 6i ). The higher-resolution measurements of hair bundle heights that we made using SEM stereoimaging showed that distal HCs in citral-treated BPs developed hair bundles that averaged just 62.7% of the mean height of bundles in the distal half of the control cultures ( P< 0.05, n BPs =4, Fig. 7 ). As an additional means of examining cellular responses to RA signalling, we cultured E6.5 BPs in medium containing 10 μM BMS 493, which antagonizes RA signalling by strongly enhancing nuclear corepressor binding to RARs [36] . In BMS 493-treated cultures, distal HCs formed luminal surfaces that were 43% larger ( P <0.05, n BPs =6, Fig. 6i ) and hair bundles that were 71.3% of the mean hair bundle height that developed in distal HCs of controls ( P <0.05, n BPs =6, Fig. 6j ). To rule out the possibility that the exogenous RA might have prevented differentiation of HCs at the proximal end of the cultured BPs or that the citral treatments might have prevented differentiation of HCs at the distal end, we immunostained BPs with the HCS-1 antibody and Alexa Fluor 488-phalloidin, then used ImageJ (NIH) to count hair bundles and HCS-1+ HC somata that differentiated under those conditions. The counts showed that BPs cultured in control medium developed 8,478±196 HCs (mean±s.e.m. ; n BPs =3), while BPs cultured with 500 nM RA developed 8,390±128 HCs ( n BPs =3) and those cultured with citral developed 8,511±326 HCs ( n BPs =3). Since the BPs that developed in control medium and media containing RA or citral all formed 80–85% of the ~10,500 HCs that develop in ovo [37] , it is unlikely that the effects of the RA and citral treatments result from suppression of HC differentiation. Thus, RA signalling appears to be necessary to induce the formation of distal-like HC phenotypes. Evidence of a role for RA in patterning electrical tuning Electrical tuning in reptile and avian HCs is dependent on differences in the gating kinetics of calcium-activated, large-conductance potassium (BK) channels [2] , [3] , [4] , [5] , [38] . BK channels consist of a pore-forming α subunit, encoded by Kcnma1 , and auxillary β 1 subunits, encoded by Kcnmb1 . β 1 is preferentially expressed in the low-frequency-tuned distal HCs, and appears to slow BK channel kinetics [38] , [39] , [40] , [41] . Chicken cochlear HCs express Kcnma1 as early as E11 (ref. 40 ) and exhibit functional Ca 2+ -activated K + channels by E16–E18 (ref. 41 ). Since expression of these channels is fundamental to HC frequency responses, we tested whether RA signalling would influence the development of the gradient of Kcnmb1 mRNA by establishing cultures of BPs at two stages before the onset of Kcnma1 expression. For these experiments, we placed E6.5 and E10 BPs in culture with 500 nM RA or control media for 3 days, then divided each into proximal and distal halves. We pooled samples from six BPs from each group, and measured Kcnmb1 mRNA levels using qRT–PCR. In the proximal halves of RA-treated BPs, Kcnmb1 expression was 7.9-fold higher and 17.5-fold higher than in controls at E6.5+3DIV and E10+3DIV, respectively (E6.5+3DIV: P =0.0402, Student’s t- test, n= 6; E10+3DIV: P =0.0103, Student’s t- test, n =3). In the distal halves of RA-treated BPs, Kcnmb1 expression was 4.8-fold higher than in controls at E6.5+3DIV ( P =0.0302, Student’s t- test, n= 7), but it was not significantly different between RA and control cultures in the E10+3DIV samples ( P =0.1820, Student’s t- test, n =3). Consistent with expectations, in the proximal half of the BP, where HCs exhibit faster BK channel kinetics and less expression of Kcnmb1 in ovo [5] , [6] , [39] , the RA treatments produced greater upregulation of Kcnmb1 expression (relative to controls). While in the distal half of the BP, RA treatments yielded modest, but significant increase in Kcnmb1 expression early in development (E6.5+3DIV), but did not change Kcnmb1 expression at the later time point (E10+3DIV), when RA levels are high distally ( Fig. 3 ). Local application of RA induces distal-like phenotypes To determine whether a local source of exogenous RA would cause proximal HCs to develop distal-like properties, we soaked 80–100 μm ion-exchange beads (AGIX-8, Bio-Rad) in RA or vehicle alone and implanted a single bead in the proximal end of E6.5 BPs before culturing them for 6 days. HCs that differentiated within 100 μm of the RA-soaked beads developed smaller luminal surfaces ( P =0.0013, Student’s t- test, n= 6, Supplementary Fig. 2d ) and longer hair bundles ( P =0.0015, Student’s t -test, n =6, Supplementary Fig. 2e ) than HCs that developed in similar locations adjacent to DMSO-soaked beads that were implanted in the controls. RA upregulates the expression of two actin crosslinkers The results presented above demonstrated a role for RA in the specification of stereocilia bundle length and number. To explore the potential mechanism of this regulation, expression of Espin, Fascin-2 (Fscn2), Fimbrin (Pls1) and T-plastin (Pls3), crosslinking proteins that regulate the elongation of the actin-filled stereocilia [42] , [43] , [44] , [45] , [46] , [47] was examined by qPCR following RA treatment for 3 days beginning on E6.5. Control and the RA-treated BPs showed no differences in Pls1 or Pls3 expression ( Supplementary Fig. 3 ), but mRNA levels for Espin increased 1.9-fold proximally and 2.3-fold distally in RA-treated versus control BPs. Likewise, Fscn2 expression increased 3-fold and 2.8-fold in proximal and distal halves, respectively ( Fig. 8a,b ). Since it is well established that Espin levels regulate stereocilia length [44] , [48] , we cultured BPs in RA or vehicle control media for 24 h to investigate whether brief treatments would influence its expression. This resulted in a pronounced 19.2-fold upregulation of Espin proximally and a 4.8-fold upregulation distally, compared with controls ( P <0.05 for each, Student’s t- test, n =6). The greater apparent increase in RA-induced Espin expression at the proximal end of the BP likely stems in part from the relatively low Espin expression that occurs at that location in controls, and is consistent with longitudinal differences in Espin expression onset in ovo , where distal expression precedes proximal expression by 2–3 days [49] . 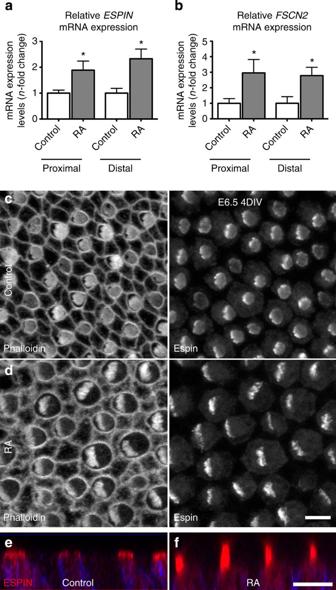Figure 8: RA treatments upregulate expression for actin crosslinking proteins expressed within stereocilia. (a) Relative mRNA expression levels forEspinin proximal and distal regions of E6.5 BPs cultured 3 days in control medium or medium supplemented with RA. Expression levels were normalized relative to the average mRNA expression in vehicle controls.Espinexpression was 1.9-fold greater in the proximal region with RA treatments (P=0.0147; Student’st-test;n=5) and 2.3-fold greater in the distal region (P=0.0079, Student’st-test;n=7). (b) Relative mRNA expression levels forFscn2in proximal and distal regions of E6.5 BPs cultured for 3 days in control medium or medium supplemented with RA. Expression levels were normalized relative to the average mRNA expression in vehicle controls.Fscn2expression was threefold greater in the proximal region with RA treatments (P=0.0295, Student’st-test;n=3) and 2.8-fold greater in the distal region (P=0.0305; Student’st-test;n=4). (c) Proximal HCs that developed in E6.5 BPs from the left ear that were cultured for 4 days in vehicle control medium, fixed and immunolabelled with Espin. Left panel shows the grey scale from Alexa Fluor-488-phalloidin labelling and the right panel shows the grey scale image from Espin labelling. HCs formed hair bundles with circular outlines. (d) Proximal HCs that developed in E6.5 BPs from the right ear that were cultured for 4 days in medium supplemented with RA. Hair bundles in these HCs formed semicircular outlines with more pronounced Espin immunofluorescence. (e,f) Images showingzaxis of Espin (red) and HCS-1 (blue) merged immunofluorescence in proximal HCs of E6.5 BPs cultured 4 for days with vehicle control (e), or with RA (f). The Espin-positive hair bundles were noticeably longer in the HCs that were exposed to exogenous RA. Graphs show mean mRNA expression levels (n-fold change) ±s.e.m. Scale bars, 5 μm. Figure 8: RA treatments upregulate expression for actin crosslinking proteins expressed within stereocilia. ( a ) Relative mRNA expression levels for Espin in proximal and distal regions of E6.5 BPs cultured 3 days in control medium or medium supplemented with RA. Expression levels were normalized relative to the average mRNA expression in vehicle controls. Espin expression was 1.9-fold greater in the proximal region with RA treatments ( P =0.0147; Student’s t- test; n =5) and 2.3-fold greater in the distal region ( P =0.0079, Student’s t- test; n =7). ( b ) Relative mRNA expression levels for Fscn2 in proximal and distal regions of E6.5 BPs cultured for 3 days in control medium or medium supplemented with RA. Expression levels were normalized relative to the average mRNA expression in vehicle controls. Fscn2 expression was threefold greater in the proximal region with RA treatments ( P =0.0295, Student’s t- test; n= 3) and 2.8-fold greater in the distal region ( P =0.0305; Student’s t- test; n =4). ( c ) Proximal HCs that developed in E6.5 BPs from the left ear that were cultured for 4 days in vehicle control medium, fixed and immunolabelled with Espin. Left panel shows the grey scale from Alexa Fluor-488-phalloidin labelling and the right panel shows the grey scale image from Espin labelling. HCs formed hair bundles with circular outlines. ( d ) Proximal HCs that developed in E6.5 BPs from the right ear that were cultured for 4 days in medium supplemented with RA. Hair bundles in these HCs formed semicircular outlines with more pronounced Espin immunofluorescence. ( e , f ) Images showing z axis of Espin (red) and HCS-1 (blue) merged immunofluorescence in proximal HCs of E6.5 BPs cultured 4 for days with vehicle control ( e ), or with RA ( f ). The Espin-positive hair bundles were noticeably longer in the HCs that were exposed to exogenous RA. Graphs show mean mRNA expression levels ( n -fold change) ±s.e.m. Scale bars, 5 μm. Full size image Ultrastructural observations have shown that differences in the onset times and the durations of phases of stereocilia elongation underlie the length gradations that develop within and among the hair bundles in the chicken BP [25] . To test whether increasing the duration of the exposure to exogenous RA would stimulate precocious elongation in proximal hair bundles, we cultured four pairs of BPs from E6.5 chicken embryos for 4 days. The BP from the right ear of each pair was cultured in RA medium and the BP from the left was cultured in control medium. When we fixed and immunolabelled the BPs for Espin, we observed that the proximal hair bundles in the control cultures were circular in outline and exhibited limited Espin expression. After 4 days in culture with exogenous RA, proximal cells in the BPs from the right ears of the same embryos developed taller, semicircular hair bundles and more pronounced Espin immunofluorescence ( Fig. 8c–e ). In ovo , E10.5 BPs have hair bundles that are circular in outline and contain uniformly short stereocilia [37] . The bundles will begin to elongate and express Espin as they progress from circular to rectangular outlines between E10–E12 (refs 27 , 49 ). Since the bundles in the proximal halves of the RA-treated BPs exhibit characteristics that normally do not develop in ovo until E12 (ref. 8 ), these findings raise the possibility that the 4-day exposure to exogenous RA stimulated precocious development of the hair bundles. Interactions between RA and Bmp7 signalling pathways A distal-to-proximal gradient of bone morphogenetic protein 7 (Bmp7) occurs in BPs from E6.5 through post-hatch ages [50] . In other systems, RA can act as either an inhibitor or an activator of Bmp7 expression [51] , [52] , so we investigated whether RA signalling would influence the Bmp7 gradient. For this, we cultured groups of six E6.5 BPs in media that contained 500 nM RA, 5 μM citral or vehicle alone for 24 h and used qRT–PCR to assess Bmp7 mRNA levels in the proximal and distal halves. Bmp7 mRNA levels in proximal and distal regions of citral-treated BPs and the levels in the distal regions of RA-treated BPs did not show clear differences from controls. However, levels of Bmp7 mRNA in the proximal half of RA-treated BPs decreased to 59.9% of the levels measured in controls, suggesting that RA suppressed Bmp7 expression ( n= 10, Supplementary Fig. 4a ). To determine whether Bmp7 would have a reciprocal inhibitory effect on RA signalling, we cultured groups of six E6.5 BPs in media containing either 400 ng ml −1 Bmp7, 100 ng ml −1 noggin, a potent antagonist of Bmp and TGF-β, or vehicle alone and assessed Raldh3 mRNA. We did not detect differences in Raldh3 expression levels between the proximal and distal halves of the Bmp7-treated BPs or between the distal halves of noggin-treated BPs and distal halves of controls, but the noggin treatment increased Raldh3 mRNA 2.26-fold in the proximal end ( n= 4, Supplementary Fig. 4b ), suggesting that Bmp signalling may normally inhibit proximal Raldh3 expression at E6.5. Taken together with our RA treatment results, these data are consistent with the possibility that the longitudinal counter gradients of Bmp7 and Raldh3 expression are maintained at E6.5 through reciprocal inhibitory feedback. Since the Raldh3 expression gradient reverses between E6.5 and E10 and becomes a distal-to-proximal gradient, like the gradient of Bmp7 expression, we next tested for positive interactions of these signalling pathways at E10. For this, we cultured groups of six E10 BPs in media containing 500 nM RA, 5 μM citral or vehicle alone for 24 h and measured Bmp7 expression. There were no detectable differences in Bmp7 expression in either region of the citral-treated BPs or in the distal region of RA-treated BPs, but Bmp7 expression increased 2.96-fold in the proximal end of RA-treated BPs ( n= 5, Supplementary Fig. 4c ). While there may be a trend towards elevated Bmp7 in the distal halves of RA-treated BPs, the sampled data values were not significantly different ( P >05; ANOVA with Newman–Keuls post-test, n= 5). We then measured Raldh3 expression in E10 BPs cultured with 400 ng ml −1 Bmp7, 100 ng ml −1 noggin, or vehicle alone for 24 h. Similar to the effects of noggin at E6.5, Raldh3 mRNA increased 2.41-fold in the distal end of noggin-treated BPs. In contrast to the E6.5 BPs where Raldh3 levels were suppressed by Bmp signalling, in the E10 BPs Raldh3 expression increased 2.29-fold and 4.06-fold in the proximal and distal ends with the Bmp7 treatments ( n =7, Supplementary Fig. 4d ). In E10 BPs, the increase in Bmp7 expression after RA treatments and increased Raldh3 expression after Bmp7 treatments suggest these signalling pathways may positively reinforce their distal-to-proximal gradients at the stage when HC phenotypes differentiate. Despite the importance of tonotopic organization within auditory sensory epithelia for speech comprehension and communication, our understanding of how the phenotypic characteristics of HCs are organized at different positions along these epithelia is rudimentary. In this study RNA-seq analysis identified signalling pathways that are expressed in patterns consistent with a role in regulation of the developmental acquisition of HC phenotypes in the chicken BP. We chose to focus on RA signalling because the RNA-seq data suggested the existence of a gradient of RA along the tonotopic axis. Also, RA is known to play roles in patterning other embryonic tissues [18] , [53] , including the early embryonic otocyst that will eventually form the inner ear [16] , [29] , [30] . While our initial RNA-seq data suggested a proximal-to-distal decreasing gradient of RA at E6.5, subsequent experiments demonstrated that this gradient rapidly switches to a distal-to-proximal decreasing gradient. Moreover, the results of functional experiments indicated that the distal-to-proximal gradient seems to be the relevant gradient in terms of patterning HC phenotypes along the tonotopic axis. The significance of the proximal-to-distal Raldh3 expression gradient evident in both the RNA-seq and qPCR data at E6.5 is unclear. As our results show ( Supplementary Fig. 4 ), RA can inhibit Bmp7 signalling, so the proximally high Raldh3 expression at E6.5 may underlie RA-mediated enforcement of a distal-to-proximal gradient of Bmp7 that has been shown to exist within the BP between E6 and E8 (ref. 50 ). It is intriguing that the gradient of Raldh3 mRNA ( Fig. 1 ) reverses after E6.5 and becomes an increasingly strong distal-to-proximal gradient as HCs within the BP begin to develop location-specific phenotypes. Since HCs are the primary source of Raldh3 at E10, we hypothesize that local differences in the numbers and spatial densities of HCs may underlie the reversal. As the BP develops, its proximal end becomes narrower while the distal end becomes broad and rounded ( Fig. 1b ). This results in a marked difference in the number of HCs at each end of the BP. A transverse section through the distal end of the BP contains as many as 46 HCs, but a similar section through the much narrower proximal end contains far fewer HCs [54] . Exposure to exogenous RA caused HCs in the proximal part of the BP to develop fewer and taller stereocilia, smaller luminal surfaces and higher levels of expression of the β subunit of the BK channel These results are consistent with increased RA signalling promoting the development of a distal-like HC phenotype. Moreover, the positive effects of RA on the expression of Espin and Fscn2 , factors encoding proteins that crosslink actin filaments and are known to be expressed in developing stereocilia at levels that correlate with their eventual length [47] , [55] , suggest a potential mechanism whereby RA signalling could directly regulate the patterning of bundle morphology. Consistent with this hypothesis, studies in other systems have demonstrated that RA can induce RAR binding at Espin ’s transcriptional start site, and a consensus retinoic acid response element (RARE) has been identified within the Fscn2 promoter [56] , [57] . Finally, while stereocilia on proximal HCs cease elongating by E12 in ovo , those on distal HCs continue to elongate for the first 2 weeks post hatching [25] , [37] . Raldh3 may have a role in this extended distal stereocilia elongation since it continues to be highly expressed in the distal region of the BP through P14 ( Fig. 1d ). It has been proposed that each HC may use the same amount of F-actin when forming a hair bundle, because proximal HC bundles in the BP contain large numbers of short stereocilia, while distal HC bundles contain low numbers of much longer stereocilia [58] . If this proposal is correct, then the hair bundle phenotypes observed at different longitudinal positions along the BP might result from the utilization of a fixed cellular pool of actin that is controlled by oppositely directed signals to regulate stereocilia elongation versus number in each HC. As a result of stimulating HCs to form longer stereocilia, RA signalling, by extension, may subsequently limit the number of stereocilia that can be formed on an individual HC. The results in this and the accompanying article (Mann et al . [50] ) suggest a model in which gradients of Bmp7 and RA each play roles in patterning the development of a longitudinally ordered sequence of HC phenotypes along the chicken BP. At E6.5, a distal-to-proximal gradient of Bmp7 appears to specify overall positional identity. The role of the proximal-to-distal counter gradient of Raldh3 mRNA expression at E6.5 is unclear, but the early Raldh3 gradient could lead to suppression of Bmp7 transcription proximally, which would reinforce the distal-to-proximal gradient of Bmp7 protein. At E10, the expression of Bmp7 has decreased throughout the BP, and a distal-to-proximal gradient of Raldh3 becomes evident and strengthens through at least P14. In fact, levels of soluble RA appear to be higher distally than proximally at E10, which would be consistent with a role for RA in controlling differentiation of location-specific aspects of HC phenotypes, such as luminal surface size, bundle height, stereocilia number and some aspects of HC physiology. RA appears to regulate the stereocilia growth, in part, by upregulating the transcription of Espin and Fscn2. Embryonic basilar papilla dissection White Leghorn chicken embryos (Spafas) were incubated at 38–39 °C in a humidified chamber with turning. Embryos were removed from the shell, transferred to DMEM/F-12 at 4 °C under sterile conditions, staged according to Hamburger and Hamilton [59] , and then decapitated. Throughout the text, the embryonic age at the time of dissection is given (that is, E6.5, E8, E10 and E13), but experiments with E6.5 embryos were carried out only using embryos at stage 29, E8 at stage 34, E10 at stage 36 and E13.5 at stage 39. All subsequent dissections and harvesting were performed under aseptic conditions while the tissue was held at 4 °C on the dissection microscope. A transverse cut posterior to the midbrain and eyes was made to bisect the head, leaving the inner ears in the posterior portion. The skin, dorsal cranium and brain were removed to allow visualization of the cochlear ducts that lie in the base of the skull, projecting ventromedially. The mandible was removed and the cochlear ducts were dissected from a ventral approach using fine forceps. Connective tissues were teased away with fine forceps and the proximal attachment to the remainder of the labyrinth was cut off using a sapphire knife. The cochlear and lagena nerve branches were trimmed off using a sapphire knife and fine forceps. Organ culture Explants were cultured nerve-side-down on nucleopore filters atop stainless steel grids (Small Parts Inc., Seattle, WA, USA) in 35-mm dishes with 1 ml DMEM/F-12 containing 1% FBS, 0.25 μg ml −1 Fungizone (Invitrogen) and 10 μg ml −1 Ciprofloxacin (Bayer, Berlin, Germany). Either complete medium changes were made every 2 days or half the medium was changed every 24 h. Explants were cultured with 500 nM all- trans retinoic acid (Sigma), 5 μM citral (Sigma), 10 μM BMS 493 (Tocris Bioscience), 400 ng ml −1 Bmp7 (R&D Systems), 100 ng ml −1 Noggin (R&D Systems) or with 0.1% DMSO vehicle as a control. RNA extraction and quantitative PCR RNA was extracted using the RNAqueous kit (Ambion) according to the manufacturer’s protocol and was reverse transcribed using a High Capacity RNA-to-cDNA kit (Applied Biosystems). Quantitative PCR was performed in triplicates using a SensiMix SYBR Green and Fluorescein kit (Quantace) on a MyIQ/iCycler (Bio-Rad). The number of times each experiment was independently replicated is indicated throughout the results. Gene expression was analysed using the Real-time PCR miner algorithm [60] . Rplp0 was used as an endogenous reference (forward: 5′-GCTTTGTGTTCACCAAGGAG; reverse: 5′-GTCACATCACAGGGAGCAAT). Gene-specific primer sets were used as described for Kcnbm1 (ref. 39 ) (forward: 5′-ACATGAGCGTGGGCCAAAGGA-3′; reverse: 5′-CCCCGGCAACTCCGAGAACG-3′). Other primers used were Aldh1a2 ( Raldh2 ) (forward: 5′-AGATCCTGCCGCTCTGATGGC-3′; reverse: 5′-GCGAGCTGCTCTCACTGCCTT-3′), Aldh1a3 ( Raldh3 ) (forward: 5′-ACGGCCTCTGAGGGGTTTGGA-3′; reverse: 5′-TGCTGCCTTTGCTGCTTCCAC-3′), Espin (forward: 5′-ATCTACGTGCAGGCCAAGAA-3′; reverse: 5′-GTAGTAGTCACCTGTGCTCGG-3′), Cyp26b1 (forward: 5′-TAAGGACTACGCCGATGCAC-3′; reverse: 5′-CGAAGATGAGCTCCAGGGTG-3′), Cyp26c1 (forward: 5′-TTCTGCTGGGACTCCGTCTGGAG-3′; reverse: 5′-ATGCAGCATGTCCCGTGCTTTGA-3′), Pls1 (forward: 5′-CTCCCTGGTCGGTATTGCTG-3′; reverse: 5′-ACCCTCTCCAAGGTCTGACA-3′), Pls3 (forward: 5′-AAAAAGTTGCCAGGCACTCG-3′; reverse: 5′-AGATCGCATGGTGACAGCC-3′), Fscn2 (forward: 5′-AACGGCAGATTCGTCTCCAT-3′; reverse: 5′-GCGCCACTCGATGTCAAACA-3′), RXRg (forward: 5′-TCATTAAGTTTCCTGCGGGCT-3′; reverse: 5′-TGGATGATGGGCTCACAGAC-3′), RARa (forward: 5′-CAGAAGTGCTTCGAGGTCGG-3′; reverse: 5′-TTCGGCACGTCCTTCTTCTT-3′), RARb (forward: 5′-GTGTCAGTGCTTGTGAGGGA-3′; reverse: 5′-TGCAGTACTGGCAGCGATTT-3′) and Bmp7 (forward: 5′-TGGTCATGAGCTTCGTCAAC; reverse: 5′-CCTCTGGGATTCTGGAGAGA-3′). Next-gen sequencing RNA preparation Three samples were collected from each cochlear duct by cutting the duct into three approximately equal sized pieces to produce proximal, middle and distal pieces. Each sample contained a portion of the future tegmentum vasculosum and the basilar papilla sensory epithelium. The distal piece also contained region of the future lagena. The pieces were immediately transferred into three 1.5 ml Eppendorf tubes containing 0.5 ml Tri Reagent RT (Molecular Research Center, Inc., Cincinnati, OH, USA) and kept on ice until all pieces were collected. The samples were stored at −20 °C until further processing. Samples from each section of the basillar papilla were processed using Illumina mRNA-seq or TrueSeq preparation kits. Separate biological replicates were also prepared and similarly analysed. In brief, mRNA was selected by oligo-dT magnetic beads and fragmented. First-strand cDNA was generated using random primers. Second-strand synthesis, end repair, addition of a single A base and adaptor ligation were then performed. Each RNA-seq library was DNA-sequenced using either the Illumina Genome Analyzer IIx or HiSeq 2000. RNA-Seq data analyses Raw reads in FASTQ format were aligned to the Ensembl Gallus gallus reference genome (WUGSC2.1) using Tophat v1.4.0 (ref. 61 ). The output.bam file was processed by Partek Genomics Suite v6.6 (Partek Inc., St Louis, MO, USA) to assemble reads into transcripts and estimate their abundances. A gene model data set combining Ensembl and NCBI annotations was used to generate RPKM for known genes and potential novel transcripts. Statistical significance levels were calculated by one-way ANOVA. Reads mapped to different isoforms of a given gene were combined for analysis. At least one region of the basilla papilla (proximal, middle or distal) was required to be ⩾ 0.5 RPKM. A fold change of ⩾ 2 was imposed for the comparison between distal and proximal regions. An additional filter was imposed where middle samples had to exhibit RPKM values intermediate between the two ends of the basilla papilla in order to selectively capture transcripts that exhibit a gradient between the two ends. Gene lists from clustering analysis were uploaded to g:Profiler and analysed by gene group functional profiling [22] . Pathways that were predicted from g:Profilers database of literature-supported interaction data sets were visualized by Cytoscape [62] . Ingenuity pathway analysis IPA was performed to discover potential upstream activators. Supplementary Data 2 , which contains both the list of genes that are differentially expressed between the E6.5 proximal and distal thirds of the cochlea and the fold-change difference in those genes that are expressed between the proximal and distal ends, were uploaded to IPA. The IPA Upstream Regulator analytic was then performed, which generated a list of 747 potential upstream transcriptional regulators that may be involved in establishing the differences in gene expression between the proximal and distal ends of the E6.5 BP. Potential regulators were ranked based upon absolute activation Z scores, and the top 10 most significant potential regulators are shown in Supplementary Table 1 . Retinoic acid reporter cell line The RARE reporter cell line F9-RARE-LacZ, which has a RARE driving LacZ expression, was obtained from Tuanlian Luo (Harvard University) [28] . Cells were grown to confluence in 0.1% gelatin-coated 24-well plates in DMEM/F-12 containing 10% FBS, 0.5 mg ml −1 G418, 0.25 μg ml −1 Fungizone and 10 μg ml −1 Ciprofloxacin. Immediately before co-culturing with cochlea, the medium was changed to DMEM/F-12 containing 1% FBS, 0.25 μg ml −1 Fungizone and 10 μg ml −1 Ciprofloxacin. E10 cochleae were dissected, the tegmentum vasculosum was carefully removed with fine forceps and the nerve was trimmed with a sapphire blade. The lagena maculae were then cut away using a sapphire blade and the non-sensory regions of the cochlea were trimmed close to the sensory epithelium. BPs were then cut in half to produce proximal and distal segments. Retinal tissue from E10 embryos was also isolated and used as a positive control tissue. Proximal and distal cochlea segments and retina epithelium were plated on top of the reporter cells and maintained at 37 °C. RARE-LacZ cells in some wells were exposed to media that were supplemented with 5 nM RA or 100 nM RA. After 12 h in culture, the samples were fixed in 1% glutaraldehyde in 0.1 M PBS for 15 min at room temperature (RT), washed three times with 0.1 M PBS containing 0.1% deoxycholate, 0.2% NP-40 and 2 mM MgCl 2 , and then X-Gal-stained overnight at 37 °C (1 mg ml −1 5-bromo-4-chloro-3-indolyl-β-D-galacto-pyranoside with 5 mM potassium ferricyanide and 5 mM potassium ferrocyanide at pH 7.3 in 0.1 M PBS and with 0.1% deoxycholate, 0.2% NP-40 and 2 mM MgCl 2 ). Bright-field images were acquired using an Olympus SZX12 stereomicroscope. Immunohistochemistry The primary antibodies used were rabbit anti-Raldh3 (Aldh1a3; Abgent), rabbit anti-pan-Espin (generous gift from Dr James Bartles, Northwestern University), rabbit anti-RXR-gamma (Abgent) and the monoclonal antibody HCS-1. Rabbit anti-RFP (Rockland Immunochemicals) was used as a negative control. The RXR-gamma, HCS-1 and Espin antibodies recognize those antigens in chicken tissue. The Raldh3 antibody was tested via western blotting of chicken kidney tissue and it labelled a band at 56 kDa, the expected size for Raldh3 protein ( Fig. 1f ). Explants were fixed in 4% paraformaldehyde in PBS for 25 min at room temperature. Then, the tegmentum vasculosum and the tectorial membrane were removed. Samples were then blocked at RT for 1 h in PBS/0.02% Triton X-100 (PBST) containing 10% normal goat serum (Vector Laboratories), then incubated overnight in primary antibodies, followed by incubation with Alexa Fluor-conjugated secondary antibodies (Invitrogen). Samples were mounted in SlowFade (Invitrogen) and images were taken with Zeiss LSM 510 or Zeiss LSM 710 confocal microscopes. Immunoblots Eight cochleae from E6.5, E10 and E18 embryos were dissected as described above. Proximal and distal tissues were then separately pooled and analysed through immunoblotting with the rabbit antibody against Raldh3. Kidney from E18 chicken embryos was used as a positive control. Organs were homogenized in reducing SDS–PAGE sample buffer, heated to 70 °C for 15 min and microcentrifuged for 30 s to remove insoluble debris. Protein was resolved with Bis–Tris SDS–PAGE gel (Novex 4–12%, Invitrogen and TGX gels from Bio-Rad), transferred to PVDF membranes and stained with India ink. Blots were blocked in blocking buffer (ECL primer blocking reagent, GE Healthcare) for 1 h and probed with goat anti-rabbit Aldh1a3 primary antibody (Abgent; 1:1,000) in blocking buffer overnight at RT. β-actin was used as a loading control. The following day, blots were washed four times for 5 min with PBS/0.3% Tween 20, then incubated with HRP-conjugated secondary antibodies (Cell Signaling Technology) for 1 h at RT. Bands were then visualized with ECL reagent (GE Healthcare). Chemiluminescence was detected using an ImageQuant LAS4000 mini imager (GE Healthcare), and band intensity was measured and normalized against the average intensity of the actin band using ImageJ densitometry software analysis. Raldh3 levels were normalized to actin values from the same lane. Each experiment was independently analysed three times. Scanning electron microscope Immediately before fixation, the tegmentum vasculosum was carefully opened with fine forceps and the tectorial membrane was pulled away to expose the sensory epithelium. Cultures were fixed in 2.5% glutaraldehyde in 0.10 M cacodylate buffer and 2 mM CaCl 2 at pH 7.35 for 2 h at RT. After post-fixation in 1% OsO4 in the same buffer for 1 h at RT, the tissue was washed in cacodylate buffer and processed by the Osmium–Thiocarbohydrazide–Osmium method [63] . Cochleae were then dehydrated through a graded ethanol series, critical point-dried, mounted on stubs and sputter-coated with gold palladium. Samples were examined in either a JEOL 6400 or Zeiss Sigma VP HD field emission SEM. Analysis To minimize bias, all measurements relating to HC phenotype, that is, hair bundle height, stereocilia number and area of the luminal HC surface, were made in regions located midway between the superior (neural) and inferior (abneural) edges of the BP. Stereocilia number Scanning electron micrographs were used to quantify numbers of stereocilia. To characterize the HC phenotypes, we took high-magnification SEM images (~20 HCs per image) midway between the inferior (abneural) and superior (neural) edges of the BP. To avoid bias, the regions selected for analysis were chosen from a low-magnification view of the BP where HC phenotypes were not distinguishable. The extreme proximal and distal edges and the superior or inferior edges of the BP were avoided in image capture. Once regions were selected, high-magnification images were captured from three neighbouring fields in the proximal region and three neighbouring fields in the distal region (six images per BP). From each micrograph, all of the stereocilia were counted on at least three HCs. HCs that had any stereocilia blocked from view or stereocilia that were not clearly discernable were excluded. The quantification was performed blindly. One investigator took high-magnification scanning electron micrographs and then coded them. A different investigator performed the stereocilia counts without knowledge of the specific treatment or the region the micrographs were from. Stereocilia counts from the three micrographs were used to determine the average number of stereocilia that formed in HCs from proximal and distal regions of each BP. The data set was then decoded and statistically analysed using one-way ANOVA with Newman–Keuls post-test (GraphPad Prism). Hair bundle height measurements from confocal microscopy Using a 63 × 1.4 NA oil-immersion objective, we captured stacks of confocal images from the proximal and distal regions with 0.37 μm steps and a 2.0 × zoom factor. At least three images from neighbouring fields were captured at the midpoint between the superior (neural) and inferior (abneural) edges of the BP at each proximal-to-distal location. Hair bundle height was determined by measuring only the tallest stereocilia. This measurement was obtained by measuring from the middle of the base to the tip of the tallest stereocilia with the 3D Imaris software (Bitplane). Values were typically measured for eight hair bundles per image. Stereocilia lengths were then averaged from the micrographs to obtain an average length that formed in HCs from proximal and distal regions for each BP. Tests for statistical significance were conducted with GraphPad Prism 8.0. Luminal surface area HC luminal surface areas were measured from LSM 510 and LSM 710 confocal micrographs using NIH ImageJ. Tests for statistical significance were conducted with GraphPad Prism 8.0. HC counts To count the number of HCs that formed in the cultured explants, BPs that were cultured for 7 days were fixed as above and then labelled with Alexa Fluor 488-phalloidin and HCS-1. Low-magnification micrographs were taken on a Zeiss 710 confocal microscope. HCs were counted using NIH ImageJ. Hair bundle height measurements from SEM stereoimaging For an independent method of measuring stereocilia lengths, we used SEM stereoimaging [64] . E6.5 BPs were cultured in media containing 500 nM RA or 5 μM citral or 0.1% DMSO alone for 7 days, then fixed for SEM as described above. To make unbiased selections of sites in the BPs for these measurements, low-magnification images of the entire BP were taken to determine the relative positions of regions located midway between the neural and abneural edges and a distance approximately equivalent to 18% of the total length of the BP away from the distal tip and 18% of the total length of the BP away from the proximal tip. Hair bundles were viewed from behind the longest stereocilia in the hair bundle. To measure hair bundle height, stereo pairs of images were captured with 8 degrees of tilt, and height was calculated. Stereopair images from four neighbouring fields were then taken at these two regions (proximal and distal) at 15,000 × magnifications. The hair bundle heights were then analysed blindly. One individual investigator took high-magnification scanning electron micrographs and then coded them. A different investigator performed the stereocilia measurements with no information on specific treatment or which region the images were from. Stereocilia lengths were then averaged from the four micrographs to obtain an average length of stereocilia that formed in HCs from proximal and distal regions for each BP. The data set was then unblinded, quantified and statistically analysed using one-way ANOVA with Newman–Keuls post-test (GraphPad Prism). Bead implantation Anion exchange resin beads AGI-X8 (80–100 μm diameter; Bio-Rad) were washed in 100% DMSO, then soaked in either DMSO containing 0.5 mg ml −1 RA or 100% DMSO alone for 20 min at RT. Beads were then briefly washed three times in 100% DMEM/F-12 and then carefully implanted inside the proximal tip of an E6.5 BP. Implanted cochleae were cultured on stainless steel grids for 6 days, fixed with 4% PFA and stained with Alexa Fluor 488-phalloidin as described. How to cite this article: Thiede, B. R. et al . Retinoic acid signalling regulates the development of tonotopically patterned hair cells in the chicken cochlea. Nat. Commun. 5:3840 doi: 10.1038/ncomms4840 (2014).